Torque modulates nucleosome stability and facilitates H2A/H2B dimer loss The nucleosome, the fundamental packing unit of chromatin, has a distinct chirality: 147 bp of DNA are wrapped around the core histones in a left-handed, negative superhelix. It has been suggested that this chirality has functional significance, particularly in the context of the cellular processes that generate DNA supercoiling, such as transcription and replication. However, the impact of torsion on nucleosome structure and stability is largely unknown. Here we perform a detailed investigation of single nucleosome behaviour on the high-affinity 601-positioning sequence under tension and torque using the angular optical trapping technique. We find that torque has only a moderate effect on nucleosome unwrapping. In contrast, we observe a dramatic loss of H2A/H2B dimers on nucleosome disruption under positive torque, whereas (H3/H4) 2 tetramers are efficiently retained irrespective of torsion. These data indicate that torque could regulate histone exchange during transcription and replication. The nucleosome, the fundamental unit of chromatin, consists of 147 bp of DNA wrapped around a complex of histone proteins—(H3/H4) 2 tetramer and a pair of H2A/H2B dimers [1] . Nucleosomes are crucial for maintaining the genome in a compacted state, which is reflected in the high-binding affinity of the histone octamer to DNA (on the order of 40 k B T [2] , [3] ). On the other hand, nucleosomes need to provide controlled access to DNA during vital cellular processes such as transcription and replication [4] , [5] . This is accomplished via a plethora of mechanisms, including transient thermal fluctuations (breathing), nucleosome sliding, and histone loss and deposition [6] , [7] . Whole protein families, such as histone chaperones, chromatin remodelers and transcription factors, have been implicated in facilitating these transactions [7] . Recent experimental advances have also brought attention to the role that mechanical effects can have in regulating nucleosome structure and stability [2] , [8] , [9] . However, the relative importance of these factors is not clear. One of the most striking features of a nucleosome is the well-defined helical path of its DNA: ~1.65 turns are wrapped around the histone octamer in a left-handed (negative) superhelix [10] . This negative supercoiling, first discovered almost 40 years ago [11] , has been associated with nucleosome preference of negatively over positively supercoiled DNA during in vitro assembly [12] , [13] . It has also been suggested that positive supercoiling can promote nucleosome disassembly [14] , [15] . However, the physiological relevance of these observations was for a long time questioned because of the absence of evidence for unconstrained supercoiling in eukaryotes [16] . Only recently have in vivo studies convincingly demonstrated that unconstrained supercoiling is ubiquitous in eukaryotic cells, even in the presence of a full complement of topoisomerases [17] , [18] , [19] . This supercoiling was found to be transcription-dependent, in agreement with the ‘twin-supercoiled domain’ model, which states that groove-tracking enzymes, such as RNA polymerase, will generate DNA supercoiling during elongation [20] . It is therefore established that cellular chromatin can experience transient torsional stress. During RNA polymerase elongation through chromatin, nucleosomes are displaced downstream and reformed upstream; this process is often accompanied by a partial or total histone loss [21] , [22] , [23] , [24] . Because of the chiral nature of the nucleosome, transcription-generated supercoiling has been hypothesized to affect both the disruption process and the fate of histones [12] . However, the experimental evidence for such an effect has been lacking. Biochemical and single-molecule experiments have demonstrated the flexibility of nucleosomal structure under low level of torsion, but did not investigate nucleosome disruption [25] , [26] , [27] , [28] . Conversely, nucleosome ejection and reformation has been studied under the impact of force, but in the absence of torsion [2] , [29] , [30] , [31] . RNA polymerase is a powerful molecular motor, capable of exerting large forces [32] , [33] and torques [34] , [35] . To understand the consequences of its impact on the nucleosome, it is imperative to fully characterize nucleosome behaviour under mechanical stress. A comprehensive investigation of the response of a single nucleosome to force and torque requires full experimental control of a nucleosome under torsion—specifying a desired degree of DNA supercoiling at will, direct measurements of torque in the DNA and access to a large range of forces. Here we achieve these capabilities using an angular optical trap, a technique that we developed for single-molecule torsional studies [36] , [37] , [38] , [39] . By investigating nucleosome disruption under different levels of torque, we find that torque differentially affects the stability of the outer and inner turns of the nucleosome. We also observe that positive torque induced dramatic H2A/H2B dimer loss, suggesting that this could be a mechanism to regulate histone turnover during transcription. Unwrapping nucleosomes under tension and torque To probe nucleosome stability under torsion, we twisted a nucleosomal DNA molecule at low force to generate a desired degree of supercoiling, and then stretched the DNA to disrupt the nucleosome ( Fig. 1a ). The range of forces (1–30 pN) and torques (from −10 to +40 pN nm) used were chosen so as to maintain DNA in its native B-form conformation [37] , [38] , [39] , [40] and are comparable to those measured or estimated for molecular motors, such as RNA polymerase [32] , [33] , [35] . To ensure precise and efficient nucleosome positioning, we have utilized the high-affinity 601 nucleosome positioning element [41] . 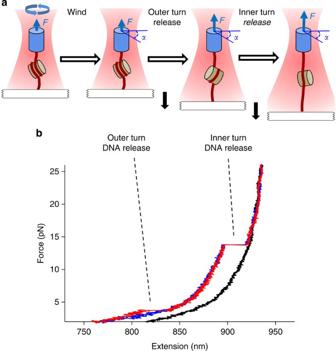Figure 1: Experimental configuration and representative traces. (a) Configuration of the nucleosome-stretching assay. DNA with a single nucleosome was torsionally constrained between a nanofabricated quartz cylinder and a coverglass, and was placed under desired torsion by adding twist via the cylinder. The angle of the cylinder,α, was then fixed, whereas the force,F, was increased at a rate of 2 pN s−1to disrupt the nucleosome. This allowed the outer and inner turns of the nucleosomal DNA to be successively unwrapped. (b) Examples of individual force-extension curves of nucleosomes under approximately +19 pN nm of torque. Red and blue curves correspond to traces with sudden or gradual outer turn DNA releases, respectively, and the black curve corresponds to a naked DNA trace. Figure 1: Experimental configuration and representative traces. ( a ) Configuration of the nucleosome-stretching assay. DNA with a single nucleosome was torsionally constrained between a nanofabricated quartz cylinder and a coverglass, and was placed under desired torsion by adding twist via the cylinder. The angle of the cylinder, α , was then fixed, whereas the force, F , was increased at a rate of 2 pN s −1 to disrupt the nucleosome. This allowed the outer and inner turns of the nucleosomal DNA to be successively unwrapped. ( b ) Examples of individual force-extension curves of nucleosomes under approximately +19 pN nm of torque. Red and blue curves correspond to traces with sudden or gradual outer turn DNA releases, respectively, and the black curve corresponds to a naked DNA trace. Full size image Figure 1b shows examples of the resulting force-extension curves. We found that DNA was released in two stages during stretching: a sudden or gradual release at low force (<6 pN); and a sudden release at high force (≥6 pN). These features resemble those of previous single-molecule studies of torsionally unconstrained nucleosomes [2] , [29] , [30] , [31] , which interpreted these two stages as the unwrapping of the outer turn DNA (low force), followed by the inner turn DNA (high force). The unwrapping process of the outer turn reflects a delicate energy balance between weaker histone–DNA interactions [8] and linker DNA bending [30] , [42] and was previously observed to proceed in either a gradual [2] , [30] or an abrupt [30] , [43] manner, depending on the buffer conditions and type of histones used. The apparent gradual unwrapping of the outer turn might also be indicative of the possibility that the release of the two halves of the outer turn is non-cooperative. In contrast, inner turn unwrapping always manifests itself as a sudden high-force transition [2] , [29] , [30] , [31] . Torque modulates outer and inner turn disruption forces Although qualitative features of nucleosome unwrapping under torque and force resembled those observed under force alone, we found significant torque-dependent quantitative differences. To characterize the effect of torque on nucleosome stability, we analysed the following parameters of the unwrapping process: amount of DNA released during the sudden disruptions, force of the outer and inner turn disruptions and the probability of sudden outer turn release. Analysis of the sudden outer and inner turn DNA release of a nucleosome indicated that, independent of torque, approximately the same amount of DNA was released in both cases ( Fig. 2a ). This indicates that, at the start of the stretching, ~140–150 bp were associated with a nucleosome on either relaxed or supercoiled DNA. 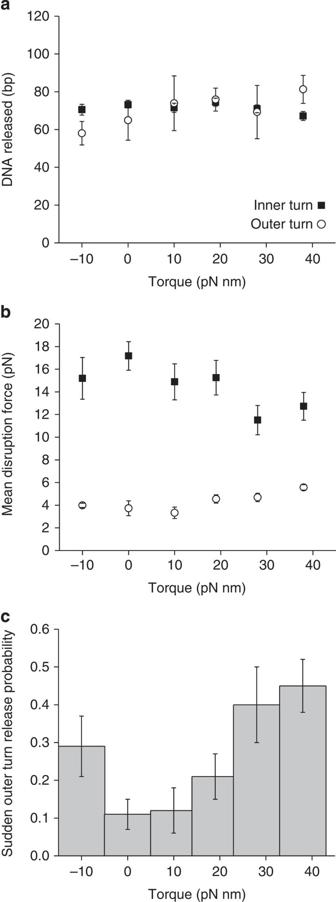Figure 2: Characterizing nucleosome disruption under force and torque. (a) Sudden release of the inner (filled squares) and outer (open circles) turns of DNA in a nucleosome. Error bars are s.e.m. (b) Mean disruption forces of the inner (filled squares) and outer (open circles) turns of DNA in a nucleosome. Error bars are s.e.m. Between 25 and 64 replicates have been obtained for each torque (Table 1). (c) Fraction of traces that displayed a sudden outer turn release as a function of torque. Error bars are s.e. of the binomial distribution (see Methods). Figure 2: Characterizing nucleosome disruption under force and torque. ( a ) Sudden release of the inner (filled squares) and outer (open circles) turns of DNA in a nucleosome. Error bars are s.e.m. ( b ) Mean disruption forces of the inner (filled squares) and outer (open circles) turns of DNA in a nucleosome. Error bars are s.e.m. Between 25 and 64 replicates have been obtained for each torque ( Table 1 ). ( c ) Fraction of traces that displayed a sudden outer turn release as a function of torque. Error bars are s.e. of the binomial distribution (see Methods). Full size image In contrast, the disruption forces were affected by torque. The trends observed were different for the outer and inner turns: torsion was found to stabilize the outer turn but destabilize the inner turn ( Fig. 2b ). The increased stability of the outer turn is consistent with the model of nucleosome under torsion proposed by Prunell and co-workers [25] , [27] , [28] , where both negative and positive torque promote tighter wrapping of the linker DNA around the histone core, thus resisting unwrapping. This tightening can disfavour DNA breathing and restrict the access of transcription factors to the nucleosomal DNA [44] . It is the inner turn interactions, however, that form the key impediment to the progression of transcription machinery through a nucleosome [8] , [23] . The decreased stability of the nucleosome inner turn observed under positive torque in our experiments suggests that torque is capable of assisting transcription. Interestingly, the magnitude of the destabilization was comparable to that of extensive histone tail acetylation [29] , known to be a hallmark of transcriptionally active chromatin [45] . We also examined the probability of observing a sudden outer turn transition as a function of torque ( Fig. 2c ). The probability exhibited a strong torque dependence, which agreed with the trends in outer turn disruption force ( Fig. 2b ). Although only ~10% of traces exhibited a sudden low-force transition for unconstrained nucleosomal DNA, this number went up to 30% for DNA under −10 pN nm and to almost 50% under +38 pN nm of torque. This provides further support to our conclusion that torque (both positive and negative) tightens the outer turn of the nucleosomal DNA. Tetrasomes do not display outer turn disruption Which histone–DNA interactions are correlated with the outer turn unwrapping? Examination of the crystal structure indicates that although H2A/H2B-DNA contacts form the bulk of those interactions, the terminus of the nucleosomal DNA superhelix is bound to the αN helix of the histone H3 (ref. 1 ). To examine the relative significance of these two contributions, we performed stretching experiments at several values of torque on tetrasomes—particles containing only an (H3/H4) 2 tetramer ( Fig. 3 ). We have compared the behaviour of recombinant Xenopus tetramers with that of the recombinant Xenopus octamers, as well as HeLa octamers ( Fig. 4 ). Even at +38 pN nm of torque, no sudden outer turn disruption was observed for tetrasomes ( Fig. 4c ), which leads us to conclude that the presence of H2A/H2B dimers is indeed required for this transition in the nucleosome and that the αN helix in histone H3 probably does not organize the last turn of DNA in the absence of H2A-H2B dimer. Notably, the high-force transition for tetramers exhibited characteristics similar to that of the octamers, indicating that this transition is predominantly governed by H3/H4–DNA interactions under our experimental conditions ( Fig. 4a,b ). 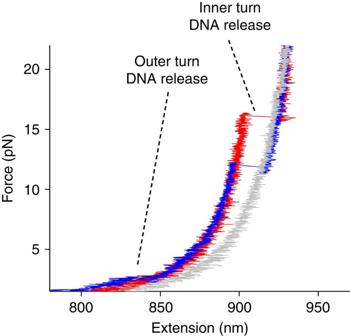Figure 3: Tetrasome force-extension curves. Naked DNA (grey), recombinant tetrasome (red), recombinant nucleosome with a sudden lower force disruption (blue), all stretched under no torsion. Figure 3: Tetrasome force-extension curves. Naked DNA (grey), recombinant tetrasome (red), recombinant nucleosome with a sudden lower force disruption (blue), all stretched under no torsion. 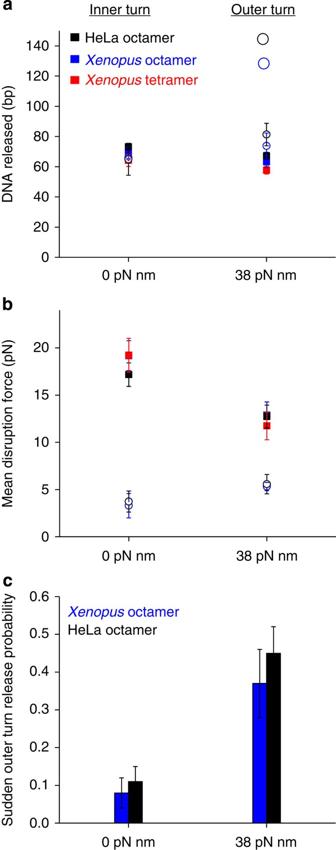Figure 4: Characterizing tetrasome disruption under force and torque. (a) Sudden release of the inner (filled squares) and outer (open circles) turns of DNA in a tetrasome and a nucleosome. Error bars are s.e.m. (b) Mean disruption forces of the inner (filled squares) and outer (open circles) turns of DNA in a tetrasome and a nucleosome. Error bars are s.e.m. Between 15 and 37 replicates have been obtained for each torque (Table 1). (c) Fraction of traces that displayed a sudden outer turn release as a function of torque. Red colour refers toXenopus-recombinant tetrasome, blue refers toXenopus-recombinant nucleosome and black refers to HeLa-purified nucleosome. Error bars are s.e. of the binomial distribution (see Methods). Full size image Figure 4: Characterizing tetrasome disruption under force and torque. ( a ) Sudden release of the inner (filled squares) and outer (open circles) turns of DNA in a tetrasome and a nucleosome. Error bars are s.e.m. ( b ) Mean disruption forces of the inner (filled squares) and outer (open circles) turns of DNA in a tetrasome and a nucleosome. Error bars are s.e.m. Between 15 and 37 replicates have been obtained for each torque ( Table 1 ). ( c ) Fraction of traces that displayed a sudden outer turn release as a function of torque. Red colour refers to Xenopus- recombinant tetrasome, blue refers to Xenopus- recombinant nucleosome and black refers to HeLa-purified nucleosome. Error bars are s.e. of the binomial distribution (see Methods). Full size image Positive torque promotes H2A/H2B dimer loss Having established that outer turn unwrapping serves as an indicator of the H2A/H2B presence, we employed this observation to study the fate of histones on nucleosome disruption. In the experiment, designed to mimic effects of transcription through chromatin under torque, we first stretched the DNA under a certain torque, then relaxed the molecule, wound it to reach +38 pN nm of torque and stretched again ( Fig. 5a ). The second stretch was designed to see which histones remained bound to the DNA, and was based on the following two observations. First, the occurrence of the sudden low-force outer turn disruption requires the presence of a full octamer with both a (H3/H4) 2 tetramer and H2A/H2B dimers ( Fig. 4c ). This sudden disruption occurs at a well-defined probability for a given torque value ( Fig. 2c ) and is always followed by a high-force sudden disruption of the inner turn DNA. Second, the occurrence of a sudden high-force disruption requires the presence of only the (H3/H4) 2 tetramer ( Fig. 4 ), and represents the sudden unwrapping of the inner turn DNA for a nucleosome or the sudden unwrapping of a single turn of a tetrasome. This always occurs as long as a (H3/H4) 2 tetramer is present. The torque for the control stretch (+38 pN nm) was chosen because it had the largest chance of observing a sudden low-force transition ( Fig. 2c ). 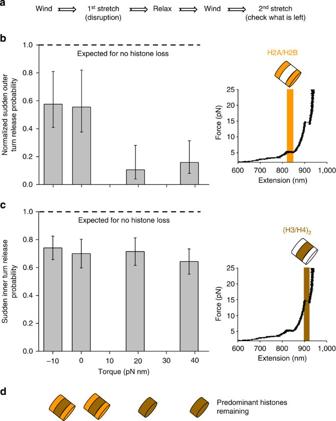Figure 5: Histone fate on disruption under torque. (a) Experimental strategy to examine the nucleosome stability under torque. A nucleosomal DNA molecule was supercoiled to a desired torsion, stretched at 2 pN s−1from 1 pN up to 30 pN of force to disrupt the nucleosome before being relaxed over 1 s to 0.7 pN. It was then wound to +38 pN nm and stretched again to determine which histones remained on the DNA. The time between relaxation and the second stretching was always kept at 30 s. (b) The probability of observing a sudden disruption at low force during the second stretch (right inset) was normalized to the corresponding value of the control stretch at +38 pN nm of torque. Normalized probability of observing a sudden low-force disruption is equivalent to the probability of retaining H2A/H2B after the initial stretch. Between 21 and 28 replicates have been obtained for each torque value (Table 1). Error bars are s.e. of the ratio of two binomial distributions (see Methods). (c) The probability of observing a sudden high-force disruption (right inset) signifies the probability of retaining (H3/H4)2after the initial stretch. Between 21 and 28 replicates have been obtained for each torque (Table 1) Insets show a representative trace of the force-extension curve resulting from a second stretch. Error bars are s.e. of the binomial distribution (see Methods). (d) Cartoons of predominant histones remaining on the DNA after disruption. Figure 5: Histone fate on disruption under torque. ( a ) Experimental strategy to examine the nucleosome stability under torque. A nucleosomal DNA molecule was supercoiled to a desired torsion, stretched at 2 pN s −1 from 1 pN up to 30 pN of force to disrupt the nucleosome before being relaxed over 1 s to 0.7 pN. It was then wound to +38 pN nm and stretched again to determine which histones remained on the DNA. The time between relaxation and the second stretching was always kept at 30 s. ( b ) The probability of observing a sudden disruption at low force during the second stretch (right inset) was normalized to the corresponding value of the control stretch at +38 pN nm of torque. Normalized probability of observing a sudden low-force disruption is equivalent to the probability of retaining H2A/H2B after the initial stretch. Between 21 and 28 replicates have been obtained for each torque value ( Table 1 ). Error bars are s.e. of the ratio of two binomial distributions (see Methods). ( c ) The probability of observing a sudden high-force disruption (right inset) signifies the probability of retaining (H3/H4) 2 after the initial stretch. Between 21 and 28 replicates have been obtained for each torque ( Table 1 ) Insets show a representative trace of the force-extension curve resulting from a second stretch. Error bars are s.e. of the binomial distribution (see Methods). ( d ) Cartoons of predominant histones remaining on the DNA after disruption. Full size image Interestingly, we found that torsion differentially affected the stability of the (H3/H4) 2 tetramer and the H2A/H2B dimers within a nucleosome. High-force unwrapping on the second stretch was observed in ~70±10% of the traces, irrespective of torsion. This signifies that the (H3/H4) 2 tetramer was efficiently retained on both relaxed and supercoiled DNA ( Fig. 5c ). This lack of torque dependence can be explained by the flexible chirality of the tetramer, which can readily flip between left- and right-handed conformations [46] . For a nucleosome on relaxed or negatively supercoiled DNA, the sudden low-force disruption on the second stretch was observed at ~60±15% of that expected for a full complement of histones. This indicates that, under these conditions, a full nucleosome is retained on the DNA with ~60% probability. In contrast, the disruption of a nucleosome under positive torque caused a significant loss of H2A/H2B dimers, so that only 10–15% of the nucleosomes retained a full complement of histones ( Fig. 5b ). This observation suggests that transcription-generated positive supercoiling may result in preferential expulsion of H2A/H2B dimers ( Fig. 5d ). In this work, we present the first comprehensive investigation of single nucleosome response to torsion, examining its impact on both nucleosome stability and histone fate. We find that nucleosomes under torque and force behave qualitatively similar to nucleosomes under force alone. However, important quantitative differences suggest ways in which torque can act as an in vivo regulatory mechanism. First, torque was found to stabilize the outer turn of the nucleosome. It is known that DNA at the nucleosome entry/exit sites is prone to spontaneous unwrapping [44] , [47] , which may facilitate transcription factor binding [7] . In this scenario, torque seems to have a repressing role. The effect is expected to be subtle, and careful in vivo studies are required to evaluate its significance. On the other hand, the destabilizing effect of torque (especially positive torque) on the highly stable interactions of the nucleosome inner turn should favour transcription elongation through chromatin. We found that moderate positive torque of 10–20 pN nm, the range accessible to RNA polymerase [35] , destabilized the inner turn interactions by over 10%, an effect comparable to that of histone tail acetylation [29] . One can roughly estimate the destabilizing effect of torque on the unwrapping force of the inner turn DNA, by assuming a one-to-one correspondence between force and torque F Δ x = τ Δ θ . Given the DNA release of Δ x =25 nm and corresponding angle change of Δ θ =0.65 2 π rad (assuming a left-handed tetramer is remaining on the DNA [46] ), one expects +38 pN nm of torque to reduce the disruption force by ~6 pN, which agrees with our measurements within their uncertainty. However, one should keep in mind that this estimate is very approximate, and does not take into account the DNA geometry, the non-equilibrium nature of the process and potential histone rearrangements. Further theoretical work is needed to address this issue in a more rigorous fashion. Although the effect of torque on nucleosome disruption is relatively modest, its impact on the fate of histones on nucleosome disruption is profound. We discovered that torsion differentially influences tetramer and dimer reformation. In our experiments, the (H3/H4) 2 tetramer was efficiently retained on the DNA irrespective of torsion (~70% of the time), and the H2A/H2B dimers displayed a similar retention rate for relaxed and negatively supercoiled DNA. In contrast, moderate and high positive torsion led to almost complete (~80%) dimer loss. The moderate torque used in our experiments is within the range accessible to RNA polymerase and is therefore physiologically relevant. The dramatic dimer loss observed in our study thus suggests that torsion can provide an efficient mechanism for dimer eviction during transcription ( Fig. 6 ). Importantly, previous in vitro transcription studies on unconstrained DNA showed dimer loss only under a very high-salt concentration (300 mM NaCl) [21] , [48] or during rapid elongation [24] . Thus, the high positive torsion employed in our study seems to induce a similar effect as that of the high-salt concentration or rapid elongation in destabilizing a nucleosome and inducing dimer loss on transcription. 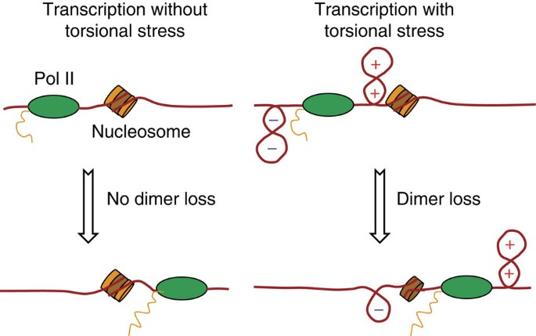Figure 6: A cartoon illustrating RNA polymerase II elongation through chromatin. During transcription under low torsion, nucleosomes remain largely intact after transcription. In contrast, during transcription under high torsion, significant dimer loss occurs in nucleosome after transcription. (H3/H4)2tetramer is shown in brown and H2A/H2B dimer in orange. Figure 6: A cartoon illustrating RNA polymerase II elongation through chromatin. During transcription under low torsion, nucleosomes remain largely intact after transcription. In contrast, during transcription under high torsion, significant dimer loss occurs in nucleosome after transcription. (H3/H4) 2 tetramer is shown in brown and H2A/H2B dimer in orange. Full size image In this work, we have used nucleosomes assembled on the high-affinity 601-positioning element. It has been previously shown that the enhanced stability of this sequence is primarily due to the histone–DNA interactions at the dyad [49] . It is therefore expected that varying the sequence will have a primary effect on the unwrapping behaviour of the nucleosome inner turn. Indeed, stretching experiments by Gemmen et al . [50] have demonstrated increased variability in the inner turn unwrapping force for nucleosomes assembled on heterogeneous DNA. However, the qualitative trends in the torque dependence of the unwrapping force observed here should hold for any sequence. Moreover, as the stability of the outer turn is not significantly enhanced by the 601 sequence [49] , we believe that our observations of H2A/H2B loss are likely to be generalizable to other sequences. Our experiments are aimed at mimicking the processes of transcription and replication, which require the complete unwrapping of the nucleosomal DNA. It is conceivable that in other instances nucleosomes can be subjected to lower stress, sufficient only to disrupt the outer turn interactions. It would be of interest in future studies to explore the effect of torque on the dimer loss in those cases. Previous in vivo studies found that H2A/H2B dimers are quickly exchanged at sites of active transcription [51] . This may have functional significance for the deposition of histone variants (such as H2A.Z) that are known to regulate transcription [52] . Although many histone chaperones and remodelers, such as Nap-1, FACT, RSC and others, have been implicated in assisting H2A/H2B disassembly [52] , our study suggests that transcription-generated supercoiling alone can lead to efficient dimer removal. The plausibility of such a mechanism is supported by recent observations of association between active transcription and DNA supercoiling in vivo [17] , [18] . Importantly, the observed stability of tetramers in our study is also in agreement with in vivo observations of the slow exchange of H3/H4 histones [51] . In summary, we propose that, on the level of individual nucleosomes, torque primarily acts as a regulator of histone exchange. Specifically, positive torsion encourages H2A/H2B dimer eviction. More work is needed to investigate the relationship between transcription-generated dynamic supercoiling and histone loss and replacement in vivo . DNA construct The DNA construct used for all experiments consisted of four pieces: two middle segments and two linker segments. Linkers were made by performing PCR on the pLB601 plasmid [38] with a mix of 0.2 mM unmodified dNTPs (Roche Applied Science) and 0.08 mM biotin-16-dCTP (Chemcyte Inc.) or 0.04 mM digoxigenin-11-dUTP (Roche Applied Science). For biotin-modified linkers, the primers used were 5′-TCC AGC CAA GAG ACC AGC CGG AAG CAT AAA-3′ and 5′-CGA AGG GAG AAA GGC GGA CAG-3′; for dig-modified linkers: 5′-TCC ACG GTA GAG ACC AGC CGG AAG CAT AAA-3′ and 5′-CGA AGG GAG AAA GGC GGA CAG-3′. Resulting 535 bp DNA fragments with multiple tags were digested with Bsa I (New England Biolabs) to create single 4-bp overhangs and purified (PureLink Quick PCR Purification Kit, Invitrogen). Middle segments (1,058 and 1,720 bp) were created by PCR from the pLB601 and pBR322 (New England Biolabs) plasmids, respectively, and then were digested with Bsa I to create two 4-bp overhangs and purified. The following primers were used: 5′-ATG GGC GAA ATC TGA CGA GAC CCA GAC AAC G-3′ and 5′-CCG CCA TTT GGC CGA GAC CAC GGA TAC-3′ for the 1-kb segment; 5′-CAA TGA TAC CGC GAG ACC CAC GCT C-3′ and 5′-GCT CTG CCT CAG CGA GAC CTA CGA GTT GC-3′ for the 1.7-kb segment. The shorter (1 kb) segment contained the 601-positioning element [53] in the middle and was used for nucleosome assembly. All the Bsa I cut sites were introduced via PCR primers. Nucleosome assembly We used purified HeLa histones, which were assembled into nucleosomes using a well-established salt-dialysis method [54] . Briefly, core histones were first mixed with the DNA segment containing 601-positioning element in the assembly buffer (final concentration 2 M NaCl, 20 mM Tris pH 7.5, 1 mM EDTA, 10 mM dithiothreitol (DTT), 0.1 g l −1 acetylated BSA). For each reconstitution, several histone-DNA ratios were used so that the most efficiently reconstituted template could be selected. The solution was then transferred into custom-made dialysis chambers. The latter were placed into high-salt buffer (2 M NaCl, 10 mM Tris pH 7.5, 1 mM EDTA, 1 mM DTT, 0.2 g l −1 sodium azide). This solution was dialysed against low-salt buffer (200 mM NaCl,10 mM Tris pH 7.5, 1 mM EDTA, 1 mM DTT, 0.2 g l −1 sodium azide) at 1 ml min −1 for ~24 h. Afterwards, the samples were transferred to zero-salt buffer (10 mM Tris pH 7.5, 1 mM EDTA, 1 mM DTT) to equilibrate. Nucleosomes were stored at 4 °C for several weeks. For tetrasome experiments, recombinant Xenopus laevis (H3/H4) 2 tetramers were used. To control for potential differences between different types of histones, we also assembled nucleosomes using recombinant Xenopus laevis octamers with the same protocols, and performed experiments using these nucleosomes. Single-molecule experiments On the day of the experiment, the four DNA pieces (including 1 kb fragment with a single-assembled nucleosome or tetrasome) were mixed in equal ratios at 5–10 nM concentration (25 nM for tetrasome experiments) and ligated at 16 °C for 1 h. Experiments were conducted in a climate-controlled room at a temperature of 23±1 °C in a nucleosome buffer containing 10 mM Tris-Cl (pH 8.0), 100 mM NaCl, 1.5 mM MgCl 2 , 1 mM EDTA, 1 mM DTT, 0.02% Tween and 2 mg ml −1 acetylated BSA. Casein from bovine milk (Sigma) at 4 mg ml −1 was used to passivate the surface. To verify that all histones were present under our buffer conditions, we have performed unzipping experiments [8] , [55] , [56] . The DNA construct for these experiments consisted of two separate segments. An ~1.1-kbp anchoring segment was prepared by PCR from the plasmid pRL574 using a digoxigenin-labeled primer (5′-GTT GTA AAA CGA CGG CCA GTG AAT-3′) and a reverse primer (5′-CCG TGA TCC AGA TCG TTG GTG AAC-3′) and then digested with Bst XI (New England Biolabs) to produce a ligatable overhang. The unzipping segment was prepared by PCR from the plasmid p601 by using a biotin-labeled primer (5′-ATG ATT CCA CCG ATC TGG CTT-3′/iBiodT/5′-AC ACT TTA TGC-3′) and a reverse primer (5′-AGC GGG TGT TGG CGG GTG TC-3′) and then digested with Bst XI and dephosphorylated using calf intestinal alkaline phosphatase (New England Biolabs) to introduce a nick into the final DNA template. Nucleosomes were assembled onto the unzipping fragment by the salt dialysis method as described above. The two segments were joined by ligation immediately before use. An optical trapping set-up was used to unzip single DNA molecules by moving the microscope coverslip horizontally away from the optical trap. As barriers to fork progression were encountered, a computer-controlled feedback loop increased the applied load linearly with time (15 pN s −1 ) as necessary to overcome those barriers. Canonical nucleosome signatures were observed, confirming the stability of single nucleosomes under our experimental conditions. Nucleosomal DNA-stretching experiments were performed with the constraint of a fixed degree of supercoiling σ (number of turns added/intrinsic twist): −0.019, 0, +0.015, +0.028, +0.041, +0.056. At the beginning of stretching under σ =+0.041 and +0.056, plectonemes were present in the DNA, but all the disruption events were observed outside of the plectonemic region. Although DNA torsional modulus is force dependent, at high forces (>2 pN) relevant in our experiments this force dependence is negligible [57] , so that stretching process can be approximated as occurring under nearly constant torques: −10, 0, +10, +19, +28, +38 pN nm. All stretching experiments were performed using a loading rate clamp of 2 pN s −1 . Tethers were stretched to 30 pN and held for 1 s at this force. When a second stretch was desired, the force was dropped to 0.7 pN in about 1 s. The DNA was then wound to +14.8 turns at 1 Hz and then held at a constant force (so that the total time spent at 0.7 pN was always 30 s). Subsequently, stretching was performed as described above. The number of molecules used for each experimental condition is recorded in Table 1 . Table 1 Number of experimental traces. Full size table Data analysis Data were anti-alias filtered at 1 kHz, acquired at 2 kHz and decimated with averaging to 200 Hz. All data were acquired and analysed using custom-written LabView software. Detection of sudden nucleosomal DNA releases was performed by cross-correlating a step function with the extension time series. Cross-correlation time series exhibited a sharp peak at the sudden DNA release point. The force at this time point was called the disruption force. Basepair release was quantified by calculating extension difference right after and right before the release and then converting it to number of base pairs using the Worm-Like Chain model of torsionally constrained DNA [40] , [58] . Normalized sudden outer turn release probability was calculated as the ratio , where p 1 is the probability of observing a sudden outer turn release during the second (control) stretch in the histone fate experiments (always performed at +38 pN nm), and p 1 is the default probability of observing a sudden transition under this torque (rightmost bar in Fig. 2c ). As the experimental conditions are identical for these two experiments, we interpret the ratio being <1 as evidence for H2A/H2B dimer loss. Error bar σ for the probability of outer turn release p was calculated as the s.e. of a binomial distribution: where n is the number of trials. Error bar for the normalized sudden outer turn release probability on second stretch was calculated by defining the 66% confidence interval of the ratio of two proportions: where p 1 is the sudden outer turn release probability on second stretch at +38 pN nm, p 2 is the sudden outer turn release probability on control stretch +38 pN nm, n 1 and n 2 are the respective number of trials, and x 1 and x 2 are the respective number of sudden outer turn releases [59] . The distribution of the disruption force and DNA release data suggested the presence of small day-to-day variations; we therefore conservatively estimated the error of the data by using the number of days when measurements were taken as the sample size. When necessary, this s.e. was further corrected using the t -statistic to account for small number of observations ( N <10). How to cite this article: Sheinin, M.Y. et al . Torque modulates nucleosome stability and facilitates H2A/H2B dimer loss. Nat. Commun. 4:2579 doi: 10.1038/ncomms3579 (2013).